Microbial iron uptake as a mechanism for dispersing iron from deep-sea hydrothermal vents Deep-sea hydrothermal vents are a significant source of oceanic iron. Although hydrothermal iron rapidly precipitates as inorganic minerals on mixing with seawater, it can be stabilized by organic matter and dispersed more widely than previously recognized. The nature and source of this organic matter is unknown. Here we show that microbial genes involved in cellular iron uptake are highly expressed in the Guaymas Basin deep-sea hydrothermal plume. The nature of these microbial iron transporters, taken together with the low concentration of dissolved iron and abundance of particulate iron in the plume, indicates that iron minerals are the target for this microbial scavenging and uptake. Our findings indicate that cellular iron uptake is a major process in plume microbial communities and suggest new mechanisms for generating Fe–C complexes. This ‘microbial iron pump’ could represent an important mode of converting hydrothermal iron into bioavailable forms that can be dispersed throughout the oceans. Iron (Fe) is the fourth most abundant element in the Earth’s crust, but it is exceedingly rare in the oceans [1] . Fe-enrichment experiments show that Fe supply stimulates phytoplankton growth and hence the biological carbon pump, which sequesters carbon to the deep ocean [2] . Because it is such a limiting nutrient, marine microorganisms employ multiple strategies for obtaining Fe in various forms including dissolved Fe, particulate Fe (that is, minerals) and Fe tightly bound to organic complexes such as siderophores, hemophores and heme [3] . Cells transport these Fe–organic complexes through specific membrane receptors, such as TonB-dependent transporters and ATP-binding cassette (ABC) transporters, for subsequent biological utilization or storage [4] . However, an excess of Fe is toxic because of its ability to form reactive oxygen species [4] , [5] . Therefore, microbial Fe uptake is tightly controlled to maintain desirable intracellular Fe concentrations, often by the enzyme ferric-uptake regulator (Fur) [4] , [5] . Fe sequestered by bacteria in this way is responsible for a large portion of Fe acquisition by marine phytoplankton in surface oceans [6] . Mid-ocean ridge axial hydrothermal venting contributes an annual flux of 1,000–10,000 Gg of dissolved Fe to the oceans [7] . It is commonly assumed that most of this Fe is biologically inaccessible due to the rapid chemical precipitation of Fe sulfide or oxide minerals [8] . However, recent evidence suggests that organic compounds bind and stabilize Fe in hydrothermal plumes, potentially altering the fate of Fe derived from hydrothermal vents [9] , [10] , [11] , [12] , [13] , [14] . Indeed, hydrothermal Fe may be transported thousands of kilometers from the source and represents a major source of Fe to deep-ocean basins [13] , [15] , [16] . The nature and source of the organic ligands of Fe in plumes are unknown, but previous studies highlight the potential importance of microbial processes [9] , [10] , [11] . Here, to investigate the mechanisms by which microorganisms influence cycling of hydrothermal Fe, we analyze whole community gene expression (metatranscriptomics) together with Fe speciation (thermodynamic modelling and spectromicroscopy) of deep-sea hydrothermal plume (~1,950 m) and background seawater (above the plume, ~1,600 m) in the Guaymas Basin (GB), Gulf of California. We propose that the microbial uptake of iron from hydrothermal plume minerals represents a ‘microbial iron pump’ in which inorganic iron is converted into more bioavailable and mobile forms that can be dispersed throughout the oceans. 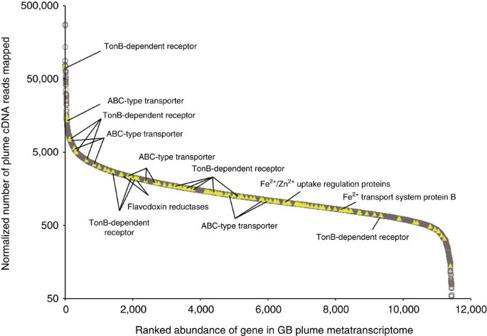Figure 1: Rank abundance of gene transcripts. The grey circles are genes of the whole GB plume community and yellow triangles are genes for Fe uptake in the plume metatranscriptomicde novoassembly. The relative abundance of gene transcripts was normalized to the length of gene fragment and the total number of all transcripts. Representative genes involving Fe transport are indicated. Microbial Fe-uptake genes in plume metatranscriptomes Shotgun sequencing of community RNA with the Illumina HiSeq-2000 platform produced 206 and 245 million short-read transcript sequences from plume and background samples, respectively ( Supplementary Table 1 ). We used a database of genes for cellular Fe uptake and utilization processes [17] , [18] to identify 28,338 transcripts of genes encoding various Fe acquisition pathways. Transcripts of Fe-related genes were more abundant in plume than background, and similar results were observed in data obtained from 454 sequencing technology ( Supplementary Fig. 1 ). The enrichment of transcripts of Fe-related genes in the plume suggests that Fe acquisition is crucial for supporting the enhanced microbial growth that occurs via chemosynthesis in deep-sea hydrothermal plumes [19] . To facilitate further analysis of these Fe-related genes, metatranscriptomic reads were assembled de novo [20] , yielding 154 different Fe-uptake genes in the plume. Several of these Fe-related genes were among the most abundantly represented genes in the entire plume metatranscriptome, including genes encoding TonB-dependent receptors and ABC-type transporters ( Fig. 1 ). Of the total Fe-related transcripts identified in the plume, nearly 77% are from just five categories, including siderophore synthesis and uptake, Fe(III) uptake, siderophore regulation and unspecified Fe transport ( Fig. 2 ). Genes for heme uptake, Fe(II) uptake, Fe storage and other biological functions were present but less abundant ( Fig. 2 ). Figure 1: Rank abundance of gene transcripts. The grey circles are genes of the whole GB plume community and yellow triangles are genes for Fe uptake in the plume metatranscriptomic de novo assembly. The relative abundance of gene transcripts was normalized to the length of gene fragment and the total number of all transcripts. Representative genes involving Fe transport are indicated. 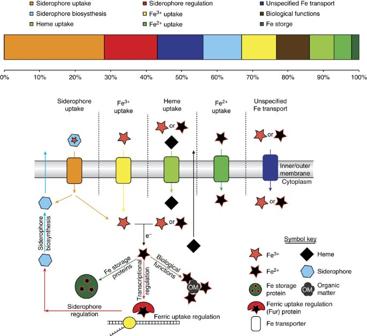Figure 2: Pathways of microbial Fe transport. The bar at the top shows the proportions of the GB hydrothermal plume transcripts assigned to each pathway, and the schematic below shows the corresponding pathways. Full size image Figure 2: Pathways of microbial Fe transport. The bar at the top shows the proportions of the GB hydrothermal plume transcripts assigned to each pathway, and the schematic below shows the corresponding pathways. Full size image Fe-related genes were further analyzed for their taxonomic affiliation using basic local alignment search tool (BLAST) searches against the non-redundant NCBI protein database. Gammaproteobacteria, primarily Alteromondaceae , Methylococcaceae and uncultured SUP05, dominated Fe-related genes in the metatranscriptome, accounting for 26–87% of transcripts from the top five pathways ( Fig. 3 ). The SAR324 group of Deltaproteobacteria also has several highly expressed genes encoding putative Fe ABC transporters, which dominate the unspecified Fe transport pathway ( Fig. 3 ). Methylococcaceae , uncultured SUP05 and SAR324 were identified previously as the major community members in the GB plume [21] . Despite the low abundance of Alteromondaceae in the GB (averaging 2.8 times coverage for metagenome and 1.01–4.04% of the total GB community at depths of 1,300–1,900 m) [20] , their Fe-uptake genes accounted for 12–45% of transcripts for the five dominant Fe-uptake pathways ( Fig. 3 ). Further analysis of the main Alteromondaceae group in the GB metatranscriptome (designated ‘GBAlt’) indicated that it was closely related to the ubiquitous particle-associated marine heterotroph Alteromonas macleodii [22] ( Supplementary Figs 2,3 ). Interestingly, GBAlt has highly transcribed genes encoding TonB-dependent and ABC transporters, including those predicted to be involved in transport of Fe siderophores or Fe-heme/hemophores ( Fig. 1 , Supplementary Fig. 4 ). Taken together, these results show that many of the dominant bacterial groups of the GB hydrothermal plume participate in cellular Fe uptake, including methanotrophs ( Methylococcaceae ), chemolithoautotrophs (SUP05 and SAR324) and heterotrophs ( Alteromondaceae ). 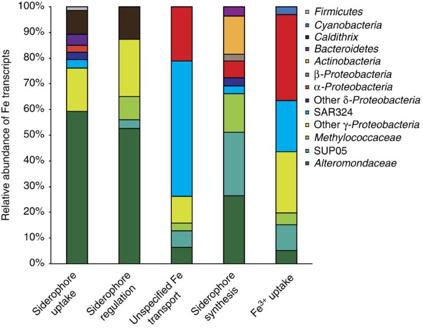Figure 3: Relative abundance of Fe transcripts from taxonomic groups. Each bar indicates the proportion of transcripts assigned to different microbial groups for the five dominant pathways of Fe uptake, respectively. Figure 3: Relative abundance of Fe transcripts from taxonomic groups. Each bar indicates the proportion of transcripts assigned to different microbial groups for the five dominant pathways of Fe uptake, respectively. Full size image More than 70% of the Fe-related transcripts we identified are involved in pathways for siderophore uptake, regulation and biosynthesis ( Fig. 2 ), indicating that siderophores are a key mechanism for microbial Fe uptake in the GB hydrothermal plume community. Siderophores are low-molecular-weight organic ligands that bind Fe(III) with high affinity and specificity. Two predominant structural classes of marine siderophores have been identified: (a) amphiphilic siderophores with fatty acid appendages of various lengths and (b) siderophores with α-hydroxy carboxylic acid moieties. The majority of siderophores identified to date are from Gammaproteobacteria and Alphaproteobacteria [23] . Our results are consistent with Gammaproteobacteria being the dominant producers of siderophores in the GB plume, accounting for 66% of Fe transcripts putatively involved in siderophores synthesis ( Fig. 3 ). Determining the molecular structure of siderophores in complex samples such as seawater is notoriously difficult [23] , [24] , [25] . The genes involved in siderophore biosynthesis, regulation and uptake identified here may provide unique insights into the nature, source and factors controlling the abundance of siderophores in plumes. However, accurate prediction of siderophore structures from genetic data is not currently feasible due to the dearth of biochemical and physiological data on the microbial groups described here, which are mostly uncultured. Siderophore production is widespread in Alteromonas species, and A. macleodii takes up siderophores but does not produce siderophores [26] , [27] , suggesting that it may utilize exogenous siderophores or other natural organic ligands. Geochemical observations and thermodynamic modelling Our metatranscriptomic data indicate that plume microorganisms obtain Fe primarily in the form of Fe(III) rather than Fe(II). This finding is consistent with previous results from geochemical modelling, which show that Fe(III) rather than Fe(II)-binding ligands are more efficient at stabilizing hydrothermal iron for transport away from the near-vent field [11] . Previous work has also shown that total Fe concentrations in end-member GB hydrothermal fluids range from 1.7 × 10 −5 to 18 × 10 −5 mol kg −1 (ref. 28 ), orders of magnitude higher than in background seawater. Given this high abundance of Fe, the prevalence of Fe-scavenging mechanisms is somewhat surprising. However, on mixing of hydrothermal fluids with seawater, much of the soluble, readily bioavailable Fe(II) precipitates as oxides and sulfides that are less bioavailable. To assess the speciation and concentration of Fe in the GB plume, we used thermodynamic modelling, X-ray absorption spectroscopy, scanning transmission X-ray microscopy (STXM) and elemental analysis by inductively coupled, plasma optical emission spectroscopy. Modelling conducted in the absence of organic ligands predicts that aqueous phase Fe(II) and Fe(III) species are at low concentration ( ca. <0.1 nmol kg −1 seawater). Measured concentrations of particulate Fe ranged from 4.15 to 15.78 nmol kg −1 seawater ( Supplementary Table 2 ). Elemental analyses also confirm the significant fraction of hydrothermal material in these samples that exhibit Al/(Al+Fe+Mn) ratios of 0.4 to below our detection limit for Al (ref. 29 ). Modelling results predict particulate Fe species including pyrite, magnetite and Fe(III) hydroxide ( Fig. 4a , Supplementary Fig. 5 ). Consistent with model predictions, Fe(III)-bearing (oxyhydr)oxide minerals such as maghemite (γ-Fe(III) 2 O 3 ), lepidocrocite (γ-Fe(III)OOH) and magnetite (Fe(II)Fe(III) 2 O 4 ) were observed by Fe 1s X-ray absorption near edge structure (XANES) spectroscopy ( Fig. 4b,c ). STXM revealed that plume particles (4–10 μm diameter range) are composed of aggregated materials that are rich in Fe as well as carbon, nitrogen and manganese ( Supplementary Figs 6 and 7 ). The C 1s XANES spectra are consistent with primarily aliphatic organic molecules having C=C (285.2 eV), -CH (287.5 eV) and O-C=O (288.7 eV) functional moieties ( Supplementary Fig. 8 ), distinct from the protein- and lipid-rich particulate organic carbon (POC) observed in plumes at the East Pacific Rise [9] , [12] . 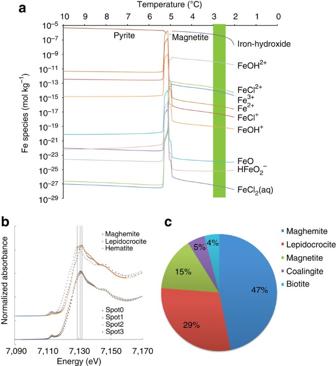Figure 4: Fe species obtained from modelling and Fe XANES spectroscopy. (a) Abundance of Fe species in mineral and aqueous phases in the GB plume (2–10 °C) predicted by the thermodynamic modelling. The temperature of the plume samples collected in this study were 2.53–2.97 °C (indicated by the green bar). (b) Fe XANES spectra of Fe-bearing minerals in plume particles and (c) their observed distribution quantified by linear combination fitting of the spectromicroscopic data. InFig. 4b, spot 0 to spot 3 are the iron XANES spectra collected from sample locations indicated inSupplementary Fig. 7a, and vertical lines at 7,129.5, 7,131 and 7,132 eV are to guide the eye; full spectra range is 7,071.4–7,367.6 eV. Figure 4: Fe species obtained from modelling and Fe XANES spectroscopy. ( a ) Abundance of Fe species in mineral and aqueous phases in the GB plume (2–10 °C) predicted by the thermodynamic modelling. The temperature of the plume samples collected in this study were 2.53–2.97 °C (indicated by the green bar). ( b ) Fe XANES spectra of Fe-bearing minerals in plume particles and ( c ) their observed distribution quantified by linear combination fitting of the spectromicroscopic data. In Fig. 4b , spot 0 to spot 3 are the iron XANES spectra collected from sample locations indicated in Supplementary Fig. 7a , and vertical lines at 7,129.5, 7,131 and 7,132 eV are to guide the eye; full spectra range is 7,071.4–7,367.6 eV. Full size image Given the prevalence of siderophore-mediated Fe(III) uptake in the GB plume microbial community and that plume Fe is expected to be predominantly in the form of particulate minerals, we propose a model for microbial acquisition of Fe through microbe–mineral interactions in hydrothermal plumes ( Fig. 5 ). Under low-dissolved Fe conditions and to support the growth that occurs in the presence of hydrothermal energy sources, microbes produce a variety of siderophores that dissolve solid-phase Fe minerals and facilitate cellular uptake [30] . Siderophore production is regulated by ferric-uptake regulator to maintain Fe homeostasis [3] . Fe(III) is reduced to Fe(II) within the cell for storage or use in biological functions in which it is complexed to a variety of intracellular organic compounds [4] . Subsequent cell death may release this organically complexed Fe into the dissolved or particulate organic carbon pool. Alternatively, because deep-sea microbial communities are thought to be relatively stable [19] , Fe that remains within cells would be widely dispersed by deep-ocean currents. In either case, these processes represent a ‘microbial Fe pump’ that mobilizes Fe bound in minerals and sequesters it within organic material where it is protected from oxidation and scavenging. This is a distinct but not mutually exclusive mechanism for plume Fe-carbon interactions compared with others that have been put forward. For example, the microbial Fe pump could generate Fe bound to POC or dissolved organic carbon (DOC) that has been observed previously [9] , [10] , [11] . An important distinction, however, is that siderophore-mediated mobilization of Fe(III) from minerals greatly expands the region in which organic complexation could take place because previous mechanisms require complexation before or immediately after Fe(II) oxidation [10] , and are thus tied to Fe(II) oxidation kinetics. In contrast, a siderophore-mediated mechanism could operate long after precipitation of Fe minerals, as plumes disperse far from hydrothermal fields. Furthermore, as siderophores produced in deep-sea hydrothermal plumes are not subjected to photodegradation, a major breakdown mechanism of siderophores in the photic zone [31] , they may disperse away from the plume and contribute to the pool of strong Fe-binding ligands (L1-type) found in the deep oceans [11] , [32] , [33] , thus enhancing the effects of ‘microbial Fe pump’ in the deep oceans. 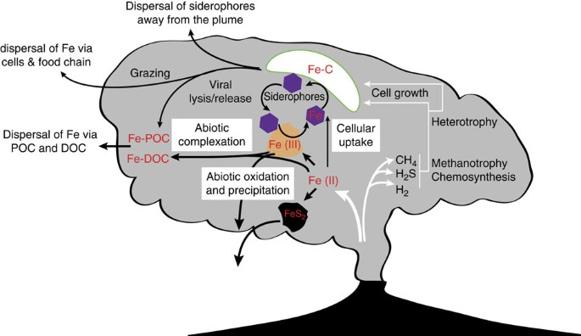Figure 5: Microbial Fe pump in deep-sea hydrothermal plumes. Uptake of Fe (primarily Fe(III)) is conducted by dominant chemosynthetic, methanotrophic and heterotrophic populations. Subsequent dispersal of Fe may occur as Fe-siderophore complexes or via whole cells or POC or DOC produced through cell lysis. Figure 5: Microbial Fe pump in deep-sea hydrothermal plumes. Uptake of Fe (primarily Fe(III)) is conducted by dominant chemosynthetic, methanotrophic and heterotrophic populations. Subsequent dispersal of Fe may occur as Fe-siderophore complexes or via whole cells or POC or DOC produced through cell lysis. Full size image The molecular and geochemical evidence presented here points to microbial scavenging of Fe from freshly precipitated minerals in hydrothermal plumes as a mechanism by which inorganic Fe is transferred to the organic phase. This process should be enhanced in deep-sea hydrothermal plumes, where microbes are stimulated by energy-rich electron donors (sulfur [34] , [35] , methane [36] , ammonia [37] and H 2 (ref. 34 )) that fuel microbial growth via autotrophy and subsequent heterotrophy ( Fig. 5 ). The few datapoints that are available suggest that the interplay between Fe, organic carbon and microorganisms is distinct at different hydrothermal systems [9] , [10] , [11] , suggesting that the fate of hydrothermal Fe in the deep sea is governed by dynamic bio-geochemical factors. Important details remain unresolved; we are currently unable to quantify the strength of this microbial Fe pump or determine the nature of the siderophores or other ligands involved. Owing to the uncultivated nature of the microbial populations discussed here, biochemical knowledge of the proteins encoded by the putative Fe-related genes is limited. However, recent evidence of extensive organically complexed Fe in dispersing hydrothermal plumes [13] , [14] highlights the need to explore these questions further. The ubiquitous and culturable nature of A. macleodii , one of the siderophore utilizers identified here, along with advances in analytical methods for probing Fe and carbon speciation in the environment, suggests that addressing such questions is within reach. Sample information Seawater samples were collected on three cruises aboard R/V New Horizon in 2004 and 2005 from the GB hydrothermal plume and background as described previously [34] , [38] . Metadata and physical/chemical characteristics of each sample are presented in detail in recent publications [21] , [34] and also listed in Supplementary Table 1 . Metatranscriptomics Nucleic acid extraction and sequencing were done as described previously [21] , [34] , [38] . The Illumina metatranscriptomic data sets from plume and background samples were used for de novo assembly, independently [20] . In brief, complementary DNA (cDNA) reads were first de-replicated by removing identical reads then quality trimmed with Sickle (score >30). These de-replicated and trimmed cDNA reads were assembled by Velvet (1.2.01) and processed using the transcriptomic assembler Oases 0.2.04 (ref. 39 ). Abundance of transcripts was determined by mapping all cDNA reads to the assembled fragments using Burrows-Wheeler Aligner (BWA) with default settings [40] and normalizing to the length of each gene. Assembled contigs were submitted to the DOE Joint Genome Institutes (JGI) Integrated Microbial Genomes website ( http://img.jgi.doe.gov/cgi-bin/w/main.cgi ) for gene calling and annotation. Identification of Fe-uptake transcripts We searched all annotated genes on assembled GB messenger RNA (mRNA) transcripts against a published Fe-uptake gene database ( E value <10 −20 ) [17] , [18] . We then compared positive hits to the non-redundant NCBI protein database. Only those that had top hits to Fe-uptake genes were considered to be involved in Fe uptake. These identified Fe-uptake genes were divided into different pathways as described previously [17] . To estimate the relative abundance of transcripts for each pathway of Fe uptake, we mapped all of the cDNA reads to each Fe-uptake gene in the GB assembly as well as available databases [17] , [18] . GBAlt analysis We searched all annotated genes on assembled GB mRNA transcripts using all of A. macleodii genes ( E value <10 −20 ) [22] . We then compared positive hits to the non-redundant NCBI protein database. Only those that had top hits to A. macleodii genes were considered to be GBAlt. Gene similarities between GBAlt and two ecotypes (ATCC 27126 and AltDE) of Alteromonas bacteria [22] were analyzed by a BLASTn analysis (bit score >50). Function of TonB-dependent transporters was predicted and classified based on the database and approach as described previously [41] , whereas classification of GBAlt ABC transporter function was analyzed based on the top hit in a BLASTx analysis. Phylogenetic relationship of GBAlt was analyzed based on the 16S ribosomal RNA (rRNA) sequence recovered by the EMIRGE program [42] from GB transcriptomes and previously published clone sequences at the same research area [38] . 16S rRNA sequences were aligned in Greengenes [43] and imported into ARB for phylogenetic analyses using maximum likelihood (RaxML) [44] . Phylogenetic trees of two housekeeping genes encoding the β-subunits of DNA gyrase ( gyrB ) and RNA polymerase ( rpoB ) were also constructed by maximum likelihood to evaluate the phylogenetic relationship of GBAlt with other ecotypes of Alteromonas bacteria [45] . Phylogenetic relationships of 16S rRNA ( Supplementary Fig. 2 ) and two housekeeping genes encoding the β subunits of DNA gyrase ( gyrB ) and RNA polymerase ( rpoB ) clearly show that the major active species of the GB plume A. macleodii population (GBAlt) are more closely related to the ‘surface ecotype’ rather than the ‘deep ecotype’ of A. macleodii ( Supplementary Fig. 2 ). Genome comparison further indicates that GBAlt (2,549 mRNAs, ~1.2 Mb) shares 95.1% average sequence identity with the surface ecotype (ATCC 27126) and 91.8% with the deep ecotype of A. macleodii (AltDE) ( Supplementary Fig. 3 ). The higher sequence similarity between GBAlt and surface ecotype demonstrates that previously observed bio-geographic distribution patterns of A. macleodii might be not be suitable for the species present at deep-sea hydrothermal vents, including GBAlt and several isolates from hydrothermal vents ( Supplementary Fig. 2 ). Thermodynamic modelling Equilibrium thermodynamic reaction path modelling was used to predict Fe-mineral precipitation, chemical concentrations and activity coefficients resulting from the mixing of seawater with GB end-member vent fluid ( Supplementary Fig. 5 ). Our approach follows those of previous studies [46] , [47] . Our Guaymas plume model was described in detail in Anantharaman et al. [34] and builds on the specific plume model implementation of Breier et al. [12] The end-member chemical concentrations and implementation used in this model are the same as that for Anantharaman et al. [34] , with the exception of a subset of assumptions that were added to more accurately predict mineral formation following our approach in Breier et al. [12] The following is a brief description of the aspects of this model pertinent to this study; interested readers are referred to Anantharaman et al. [34] for more details. The Guaymas plume reaction path is modelled through a mixing process that ends at a vent fluid to seawater dilution of 1:10,000, representing the dilution achieved at the non-buoyant plumes sampled in this study. Vent fluid composition was based on measurements made in 1982 and 2000 (refs 28 , 48 ). In situ pH was calculated from measurements of pH at 25 °C using an equilibrium reaction path model that increased the temperature of the measured fluid to the original vent fluid temperature. Background seawater dissolved O 2 concentration was based on previous measurements reported for GB hydrothermal plumes [49] . Note, the available data predate this study; actual vent chemistry during this study may have differed. Reaction path modelling was performed with REACT, part of the Geochemist’s Workbench package [50] . Conductive cooling was neglected and mixture temperatures were a strict function of conservative end-member mixing. Precipitated minerals were allowed to dissolve and their constituents to re-precipitate based on thermodynamic equilibrium constraints. Thermodynamic data were predicted by SUPCRT95 (ref. 51 ) for the temperature range of 1–425 °C (specifically 1, 25, 60, 100, 225, 290, 350 and 425 °C) and a pressure of 500 bar, a pressure and temperature range that encompasses all known deep-sea vents. SUPCRT95 uses previously published thermodynamic data for minerals, gases and aqueous species [52] , [53] , [54] , [55] , [56] . Thermodynamic data for pyrolusite, bixbyite, hausmannite, marcasite and Fe(OH) 3 were added for our study [57] , [58] . The B-dot activity model was used [59] , [60] . Temperature-dependent activity coefficients were used for aqueous CO 2 and water in an NaCl solution [50] , [61] , [62] . A general limitation of REACT is that it does not predict the thermodynamic behavior of solid solutions. Thus, minerals, such as sphalerite, pyrrhotite, chalcopyrite and isocubanite, are treated as separate phases with ideal stoichiometries. This may influence the predicted plume mineral assemblage. In Anantharaman et al. [34] , we suppressed all aqueous-phase redox couples to estimate upper-limit constraints on potential chemosynthetic metabolic energy. In this case, we use these same assumptions but because of our specific interest in Fe speciation in this study, we have added additional assumptions related to mineral formation following Breier et al. [12] The precipitation of hematite was suppressed to allow Fe hydroxide to precipitate on the basis that the latter is a closer approximation than the former to the more common amorphous Fe oxyhydroxides, which precipitate preferentially due to kinetic effects. The precipitation of Mg-bearing minerals and silicates, with the exception of amorphous silica, was also suppressed for simplicity. Some in this group have been found as minor plume constituents, others such as quartz appear kinetically inhibited; but in any case, the suppression of this group does not influence the precipitation of the minerals of interest in this study. Precipitated minerals were allowed to dissolve and their constituents to re-precipitate based on thermodynamic equilibrium constraints. Bulk elemental analysis Particulate filter samples were completely digested in 30-ml acid-cleaned perfluoroalkoxy vials (Savillex) using the following procedure based on Bowie et al. [63] The 0.2-μm, 142-mm diameter, polyethersulfone membrane filters (SUPOR, Pall Corporation) were split into 1/8 sections. Each filter split was added to a digestion vial with 2 ml of concentrated nitric acid. The vials were capped and heated at 110 °C for 4 h. After cooldown, 0.5 ml of concentrated hydrofluoric acid was added to each vial. The vials were capped and heated at 110 °C for 4 h. The vials were then uncapped and heated at 120 °C to dryness. An additional 100 μl of concentrated nitric acid was added and similarly taken to dryness to facilitate evaporation of the hydrofluoric acid. After cooldown, the digested sample was taken back into solution by adding 3 ml of a 3% nitric acid matrix. The vials were capped and heated for 1 h at 60 °C. This process resulted in the complete digestion of visible particles and in most cases the filter, in the few cases where residual filter material (<1% of the whole filter) remained it was removed by filtration of the digest solution. All acids were trace metal grade (Optima, Fisher Scientific). Vials were heated in a temperature-controlled hot plate (Qblock, Questron Technologies). Aliquots of sample digest, at a 1:10 dilution, were analyzed for Fe, Mn, Al, Ti, P, Zn, Ni, Cu and U by inductively coupled plasma optical emission spectrometry on a Varian 730-ES axial spectrometer by Activation Laboratories. External standards were used for instrument calibration. Digestion and analysis were both monitored by processing portions of the basalt geostandard BHVO-1 (ref. 64 ) with these samples ( Supplementary Table 2 ). STXM and C XANES spectroscopy STXM and C 1s X-ray absorption near edge structure (XANES) spectroscopy were performed at the Advanced Light Source, Lawrence Berkeley National Laboratory, Berkeley, CA, USA, on beamline 5.3.2.2 (ref. 65 ). GB plume particles were re-suspended from the original PES filter by gentle shaking in 0.5 ml of purified water. From this suspension, ~1 μl was deposited on a silicon nitride membrane (Silson Ltd) and air-dried. This preparation resulted in dispersed particles with no sea salt precipitates. Optical density images were made from X-ray images recorded at energies just below and at the C 1s (280, 305 eV), N 1s (395, 401.5 eV), Mn 2p (635, 643 eV) and Fe 2p (700, 709.5 eV) absorption edges. The Fe 2p 709.5 eV image will preferentially display Fe(III) if present. Fe 2p images were also collected at 707.6 eV to test the sample for Fe(II). The patterns observed for 709.5 and 707.6 eV images revealed the same pattern of Fe in the particles with differing optical densities. Therefore, only the elemental maps derived from the 709.5 eV images are displayed in Supplementary Fig. 6 . C 1s XANES spectra from regions of interest were obtained from image sequences (called stacks) collected at energies spanning the absorption edge (280–340 eV for C). Theoretical spatial and spectral resolutions were 20 nm and ±0.1 eV, respectively. All measurements were performed at ambient temperature and <1 atm He. Calibration at the C 1s edge was accomplished with the 3s (292.74 eV) and 3p (294.96 eV) Rydberg transitions of gaseous CO 2 . All STXM data processing was carried out with the IDL aXis2000 software package ( http://unicorn.mcmaster.ca/aXis2000.html ). All XANES data processing was done in program Athena . X-ray microprobe and Fe 1s XANES spectroscopy A small (~1.5 cm 2 ) portion of the original PES filter, obtained using a ceramic scalpel, was mounted on an aluminum sample holder. The remaining sample was stored frozen. Data collection at the ALS beamline 10.3.2 (ref. 66 ) had the following task flow for these filter-bound plume particles: X-ray fluorescence (XRF) mapping at multiple energies to determine the spatial distribution of elements in the particles within a region of interest; and Fe 1 s XANES spectroscopy measurements at specific locations (that is, particles or particle aggregates) within the region of interest. The distribution of Fe, Mn, Ca and other elements was measured in an area 0.995 × 1.865 mm 2 by microprobe XRF using a 7-element Ge solid-state fluorescence detector (Canberra) with a pixel size of 5 × 5 μm 2 . XRF mapping included: (1) an ‘As map’ with incident energy set to PbL 3 -50, or 12,985 eV, that provided Fe, Ni, Cu, Zn and As distributions; (2) a ‘Mn map’ with incident energy set to FeK-50, or 7,062 eV, that provided Mn distribution without interference from Fe Kα fluorescence emission; and (3) a ‘V map’ was generated by subtracting a VK-50, or 5,415 eV map from a VK+100, or 5,565 eV to distinguish V Kα from Ti Kβ fluorescence emission. Light elements, Si, S, Cl, K and Ca, were obtained from the lowest energy map collected. Individual XRF maps were deadtime corrected, aligned and channels of interest were added to a single composite map using custom beamline software [66] . The composite XRF map was used to locate particles for Fe 1s XANES spectroscopy. The monochromator energy calibration was set with the inflection point of a scan of Fe foil at 7,110.75 eV. Iron XANES were conducted in ‘quick’ mode using the fluorescence detector. Individual scans of the monochromator required 30 s, and were repeated up to 60 times. Data scans collected at the same sample location were examined for changes in line-shape and peak position, and no photon-induced sample damage was observed. Spectra were deadtime corrected, energy calibrated and averaged using custom beamline software [66] . The software program Athena was used to perform pre-edge subtraction and post-edge normalization [67] . Normalized spectra were subjected to linear combination fitting with reference spectra using custom beamline software [66] as described in previous study [12] . The Fe reference spectra database used has 94 entries [68] , [69] , [70] . Accession code s: Sequences of cDNA Illumina reads for plume and background samples of this study have been deposited in the NCBI SRA database under accession numbers SRX134769 and SRX134768 . The plume transcriptomic assembly sequences for this study have been deposited in JGI IMG/MER database under accession ID 23647000. How to cite this article: Li, M. et al. Microbial iron uptake as a mechanism for dispersing iron from deep-sea hydrothermal vents. Nat. Commun. 5:3192 doi: 10.1038/ncomms4192 (2014).